Differential regulation of theEpr3receptor coordinates membrane-restricted rhizobial colonization of root nodule primordia In Lotus japonicus , a LysM receptor kinase, EPR3, distinguishes compatible and incompatible rhizobial exopolysaccharides at the epidermis. However, the role of this recognition system in bacterial colonization of the root interior is unknown. Here we show that EPR3 advances the intracellular infection mechanism that mediates infection thread invasion of the root cortex and nodule primordia. At the cellular level, Epr3 expression delineates progression of infection threads into nodule primordia and cortical infection thread formation is impaired in epr3 mutants. Genetic dissection of this developmental coordination showed that Epr3 is integrated into the symbiosis signal transduction pathways. Further analysis showed differential expression of Epr3 in the epidermis and cortical primordia and identified key transcription factors controlling this tissue specificity. These results suggest that exopolysaccharide recognition is reiterated during the progressing infection and that EPR3 perception of compatible exopolysaccharide promotes an intracellular cortical infection mechanism maintaining bacteria enclosed in plant membranes. Endosymbioses with rhizobia enable legumes to fix atmospheric nitrogen and in return rhizobia find a niche for their growth and multiplication within legume nodules. Rhizobial infection of the model legumes Lotus japonicus ( Lotus ) and Medicago truncatula ( Medicago ) is initiated at sites where bacteria are entrapped by curled root hairs. Recent results suggest that an infection chamber is formed through remodelling of the plant cell wall before infection threads are initiated and colonized by rhizobia [1] . These plant-derived tubular structures traverse inwards to the root cortex where they ramify in nodule primordia, which are formed by associated local re-initiation of cortical root cell divisions. Finally, bacteria are released into nodule cells by endocytosis. By this process, membrane-bound organelle-like symbiosomes containing nitrogen-fixing rhizobia, in a bacteroid differentiated state, will eventually occupy most of the cytoplasmic space of infected nodule cells. This intracellular invasion mechanism contains bacteria within plant membranes from the initial invagination of the root hair membrane to the symbiosomes residing within the plant cells. Intracellular infection is, however, not the only entry mechanism found in the large and diverse legume family. Crack entry between epidermal cells, often associated with lateral root formation, is an alternative intercellular route known from a number of legumes, for example, peanut ( Arachis hypogaea ), Aeschynomene and Sesbania rostrata [2] , [3] , [4] . In some of these legumes rhizobia remain intercellular until symbiosomes are formed by endocytosis, whereas in others cortical infection threads develop from the initial infection pockets re-establishing an intracellular entry mode in the root cortex [3] . Both of these alternative crack entry pathways were also found in Lotus mutants where the normal root hair infection thread pathway was blocked, although infection efficiencies were low compared to intracellular infection via root hair infection threads [5] , [6] , [7] . Genetic analysis of loss-of-function and gain-of-function plant mutants supports the existence of two parallel, but highly synchronized, pathways controlling intracellular root hair infection and nodule organogenesis [7] , [8] . However, the plant genetic program controlling intracellular infection via infection threads remains uncharacterised. In Lotus , both root hair infection and nodule organogenesis pathways are under the control of the LysM-domain-containing Nod factor receptors, NFR1 and NFR5, that trigger two signal transduction pathways following the perception of rhizobial Nod factor signals [9] , [10] , [11] , [12] , [13] . The so-called common symbiosis pathway, shared between the rhizobial and mycorrhizal symbioses, consists of at least seven genes [14] , [15] ; a LRR receptor kinase ( SymRK ) [16] , [17] , cation channels ( Castor and Pollux ) [18] , [19] , [20] , nucleoporins ( Nup85 , Nup133 and Nena ) [21] , [22] , [23] and a calcium calmodulin-dependent protein kinase ( CCaMK ) [24] , [25] . SymRK , Castor , Pollux , Nup85 , Nup133 and Nena all act upstream of Ca 2+ spiking. Biochemical analysis suggests that NFR receptors bind Nod factor and form a complex where NFR5 interacts with SYMRK [26] , [27] , [28] . The current understanding is that this receptor activation leads to the release of calcium oscillations in the nucleoplasm [29] , [30] . Calcium oscillations are decoded by CCaMK and activated CCaMK phosphorylates CYCLOPS that acts as a transcription factor for Nin , thus promoting epidermal infection thread formation [31] , [32] . Further downstream in the organogenesis pathway the NSP1, NSP2, NIN, NF-YA1 and the AP2 type ERN1 and ERN2 transcriptional regulators are required for regulation of nodule-expressed genes and initiation of nodulation [33] , [34] , [35] , [36] , [37] , [38] , [39] , [40] , [41] . Finally, reactivation of cortical root cells resulting in nodule primordia formation is initiated by cytokinin signalling through functionally overlapping cytokinin receptors LHK1, LHK1a and LHK3 (refs 42 , 43 , 44 ). Endoreduplication involving topoisomerase ( Vag1 and SUNERGOS ) and a deubiquitination enzyme ( Amsh1 ) is also required [45] , [46] , [47] . A comparable progression of events cannot be assembled from the few components identified to contribute to infection thread development and progression. Npl1 encodes a pectate lyase presumably involved in cell wall hydrolysis [48] , Nap1 , Pir1, ArpC1 and SCARN encode proteins controlling actin rearrangement in root hairs via the SCAR/WAVE complex [49] , [50] , [51] , [52] , and a putative E3 ubiquitin ligase encoded by Cerberus is also required for infection thread development [53] , [54] . Infection threads are typically arrested in the root hair if these genes are mutated. Likewise, the transcriptional regulators CYCLOPS, NIN, NSP1 and NSP2 are required for the epidermal initiation of infection thread development. The biochemical pathway and genetic network subsequently involved in progressing infection threads into the root cortex is virtually undescribed and our understanding is mainly based on imaging. Individual plant cells initiate infection thread formation at the interface of the cell above and extend the infection thread to the interface of the cell below. Analysis of electron micrographs suggests that fusion of the infection thread wall at the site of entry into the lower cell precedes cell wall degradation and re-initiation of the infection thread in the lower cell [55] . This iterated cell autonomous process, which appears to differ from the initial infection chamber formation, advances the infection thread and, by an unknown mechanism, branching occurs in the nodule primordium before bacteria are released from the infection thread into the plant cell. Infection thread progression is synchronized and coupled to the development of primordia in a highly regulated process that has not yet been uncovered. An example of this is the abortion of most infection threads already in the epidermis. This leads to the notion of an epidermal–cortical barrier where cytokinin signalling mediates repression [56] , while endoreduplication promotes reinitiation [45] , [46] , suggesting that infection thread progression is regulated at each cell passage. Calcium oscillations observed in the plant cell just ahead of the growing infection thread suggest that Nod factor perception and CCaMK activation is involved but components of a regulatory mechanism controlling the cell autonomous advance of infection threads have not yet been identified. Here we show that perception of exopolysaccharide (EPS) synthesized by M. loti is important for maintaining an intracellular infection mode and that expression of the EPS receptor gene, Epr3 , is controlled by the symbiotic program of the plant. EPR3 acts in the root cortex and nodule primordia to support and sustain the containment of rhizobia and to facilitate an efficient infection process. EPS and EPR3 determine the cortical infection mechanism Perception of EPSs by the EPR3 receptor of wild-type Lotus (ecotype Gifu) regulates epidermal infection. epr3 mutants formed fewer root hair infection threads after inoculation with M. loti strain R7A than Gifu. Similarly, reduced root hair infection thread formation was observed after Gifu was inoculated with an EPS-deficient R7AexoB mutant [57] . To assess the role of EPS perception in later stages of the nodule infection process, we traced the consequences of perturbed EPS perception on rhizobial invasion of the root cortex and nodule primordia. The infection phenotypes of cortical nodule primordia and nodules were investigated in detail using light microscopy, confocal microscopy and transmission electron microscopy (TEM). When sections of infected nodules of R7A-inoculated epr3 plants were investigated, misguided infection threads associated with balloon-like swellings were often observed in epidermal cells, some of which reinitiated infection thread elongation into the primordia ( Fig. 1a–d ). Infection threads in Gifu plants inoculated with R7AexoB appeared thicker and seemed arrested or temporarily arrested at the cortical boundary ( Fig. 1e,f ). These observations suggest a control point for infection thread progression at the epidermal–cortical cell boundary and that EPS perception by EPR3 might be required for reinitiating infection threads at each cell passage. 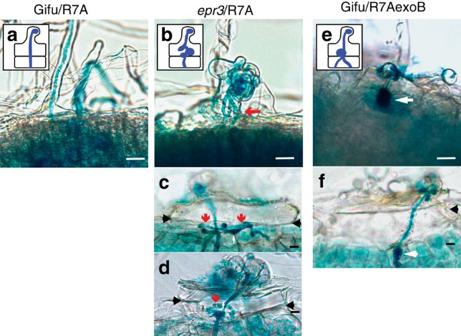Figure 1: Infection thread progression in Gifu andepr3mutants. (a) Schematic and image of infection thread targeting a nodule primordium in Gifu inoculated with R7A. (b–d) Schematic and images of misguided infection threads inepr3-9(b),epr3-10(c) andepr3-11(d) inoculated with R7A. (e,f) Schematic and images of short thick infection threads in Gifu inoculated with R7AexoB. (a–f) The behaviour of infection threads at the epidermal–cortical cell boundary in Gifu andepr3mutants inoculated with R7A or R7AexoB. Red arrows indicate misguided infection threads at the epidermal–cortical boundary (which is marked by black arrows). White arrows indicate balloon-like swellings. Scale bars, 20 μm (a–f). Figure 1: Infection thread progression in Gifu and epr3 mutants. ( a ) Schematic and image of infection thread targeting a nodule primordium in Gifu inoculated with R7A. ( b – d ) Schematic and images of misguided infection threads in epr3-9 ( b ), epr3-10 ( c ) and epr3-11 ( d ) inoculated with R7A. ( e , f ) Schematic and images of short thick infection threads in Gifu inoculated with R7AexoB. ( a – f ) The behaviour of infection threads at the epidermal–cortical cell boundary in Gifu and epr3 mutants inoculated with R7A or R7AexoB. Red arrows indicate misguided infection threads at the epidermal–cortical boundary (which is marked by black arrows). White arrows indicate balloon-like swellings. Scale bars, 20 μm ( a – f ). Full size image Corroborating these observations, we found that the highly efficient intracellular infection through infection thread progression was impaired in the epr3 mutants and intercellular bacteria were present in most nodules ( Fig. 2 ; Supplementary Fig. 1 ). At 14 and 28 days post inoculation (dpi), epr3 mutant nodules contained fewer infected cells than Gifu. Direct quantification found a significant reduction of transcellular cortical infection threads induced by R7A in epr3 nodules compared to Gifu nodules ( Fig. 2o ). Furthermore, transcellular infection threads often appeared irregular with lumpy protrusions in epr3 mutants compared with Gifu ( Fig. 2g,i,k,m ; Fig. 3a–d,i,j ). The TEM images show enlarged infection threads packed with rhizobia both between cells and within plant cells as well as intercellular bacteria ( Supplementary Fig. 1l ). In a complementary experiment where Gifu was inoculated with R7AexoB, which lacks EPS, comparable effects were observed. Intercellular infection and a reduction in cortical infection threads were characteristic for Gifu nodules induced and infected by R7AexoB ( Fig. 2j,n,o ). More detailed microscopy, focusing on infection threads and endocytosis into plant cells, revealed a release mechanism similar to the single-cell peg infections previously reported [7] ( Fig. 2n ; Fig. 3m–p ). Both the absence of EPS in R7AexoB ( Fig. 3m–p ) and inactivation of Epr3 ( Fig. 3e–l ) appear to result in plant cell invasion via this entry mode. Typically, the effects of the absence of EPS or the EPR3 receptor are fewer infected nodule cells, reduced or perturbed transcellular cortical infection threads, and rhizobia present in the intercellular space between host cells ( Fig. 2i,j,m,n ; Supplementary Fig. 1l ). These changes were even more pronounced in plants grown at 28 °C with several bacteroids enclosed within the same symbiosome membrane, which in many cases appeared to be undergoing degradation ( Supplementary Fig. 1 ). This concurs with earlier observations suggesting a role for EPS perception at the initiation of infection threads and bacterial release from infection threads [57] , [58] . 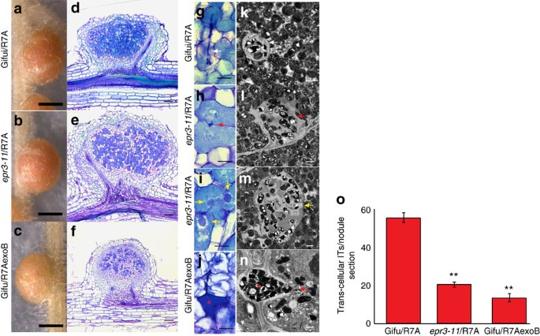Figure 2: Nodule infection phenotype in Gifu andepr3mutants. Images of intact nodules, semi-thin microscopy sections and TEM sections from Gifu inoculated with R7A (a,d,g,k),epr3-11inoculated with R7A (b,e,h,i,l,m) and Gifu inoculated with R7AexoB (c,f,j,n). Plants were grown at 21 °C and nodules sectioned 14 dpi. Light microscopy and transmission electron micrographs of sectioned nodules illustrate the infection mechanisms (g–n). White arrows indicate transcellular infection threads. Red arrows indicate peg-type intercellular infection. Yellow arrows indicate infection thread protrusions. Red stars indicate the intercellular bacteria. Scale bars, 0.5 mm (a–c); 0.1 mm (d–f), 20 μm (g–j); 1 μm (k–n). (o) Number of cortical infection threads observed in nodules at 14 days post infection (dpi). Gifu andepr3-11inoculated with R7A and Gifu inoculated with R7AexoB. Number of cortical infection threads was counted in randomly selected sections of five nodules from each combination. ** (P<0.01, Student’st-test,n=25) indicates significant difference compared to Gifu inoculated with R7A. Error bars are s.e.m. Figure 2: Nodule infection phenotype in Gifu and epr3 mutants. Images of intact nodules, semi-thin microscopy sections and TEM sections from Gifu inoculated with R7A ( a , d , g , k ), epr3-11 inoculated with R7A ( b , e , h , i , l , m ) and Gifu inoculated with R7AexoB ( c , f , j , n ). Plants were grown at 21 °C and nodules sectioned 14 dpi. Light microscopy and transmission electron micrographs of sectioned nodules illustrate the infection mechanisms ( g – n ). White arrows indicate transcellular infection threads. Red arrows indicate peg-type intercellular infection. Yellow arrows indicate infection thread protrusions. Red stars indicate the intercellular bacteria. Scale bars, 0.5 mm ( a – c ); 0.1 mm ( d – f ), 20 μm ( g – j ); 1 μm ( k – n ). ( o ) Number of cortical infection threads observed in nodules at 14 days post infection (dpi). Gifu and epr3-11 inoculated with R7A and Gifu inoculated with R7AexoB. Number of cortical infection threads was counted in randomly selected sections of five nodules from each combination. ** ( P <0.01, Student’s t -test, n =25) indicates significant difference compared to Gifu inoculated with R7A. Error bars are s.e.m. 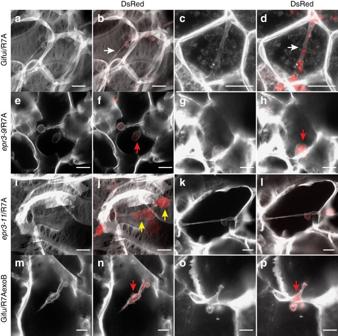Figure 3: Cortical infection threads and peg infection in Gifu andepr3mutants. Images of cortical infection threads in nodules of Gifu inoculated with R7A DsRed (a–d),epr3-9mutant inoculated with R7A DsRed (e–h),epr3-11inoculated with R7A DsRed (i–l) and Gifu inoculated with R7AexoB DsRed (m–p). At 10–14 dpi, nodules were sectioned by hand and cell walls, and infection threads were stained with 0.04% calcofluor. White arrows indicate transcellular infection threads. Red arrows indicate peg-type intercellular infection. Yellow arrows indicate infection thread protrusions. Scale bars, 10 μm. Full size image Figure 3: Cortical infection threads and peg infection in Gifu and epr3 mutants. Images of cortical infection threads in nodules of Gifu inoculated with R7A DsRed ( a – d ), epr3-9 mutant inoculated with R7A DsRed ( e – h ), epr3-11 inoculated with R7A DsRed ( i – l ) and Gifu inoculated with R7AexoB DsRed ( m – p ). At 10–14 dpi, nodules were sectioned by hand and cell walls, and infection threads were stained with 0.04% calcofluor. White arrows indicate transcellular infection threads. Red arrows indicate peg-type intercellular infection. Yellow arrows indicate infection thread protrusions. Scale bars, 10 μm. Full size image Taken together, the impaired infection of epr3 mutant nodules by R7A and Gifu nodules induced by R7AexoB indicate that EPS-mediated EPR3 signalling is required for sustaining the cortical infection thread invasion that normally mediates intracellular rhizobial infection from epidermal passage to endocytotic release into symbiosomes. The cellular Epr3 expression pattern mirrors infection Previous observations showed Epr3 promoter activation in root hairs of the susceptible zone after Nod factor perception [57] . To determine whether the suggested cortical function is reflected in the Epr3 expression pattern, we monitored Epr3 promoter activity using nuclear localized fluorescence in transformed roots expressing the pEpr3:tYFP-NLS construct. A representative root is shown in Fig. 4 covering a time span from 3 to 10 dpi after inoculation with M. loti MAFF303099. At 3 dpi, the expression was fairly uniform among root hairs. By 4 dpi, an expression focal point(s) was distinguishable above what appears to be an emerging nodule primordium. From 5 to 10 dpi, the expression in root hairs declined, while increased expression in the developing primordia abutted an area where DsRed-labelled rhizobia were observed. A similar pattern was observed using a pEpr3:GUS reporter construct ( Supplementary Fig. 2a–f ). At 7 and 14 dpi, the expression was confined to primordia and nodules, indicating organ specialization. The Epr3 promoter activity was lower and ceased in older nodules ( Supplementary Fig. 2e ). In whole mounts/sections pEpr3:tYFP-NLS expression was strong in infected epidermal cells ( Fig. 5a,b ) and in outer cortical cells immediately surrounding infection threads ( Fig. 5b ). This high level of expression appears to delineate the infection thread path from the epidermis into the outer root cortex and the nodule primordia. 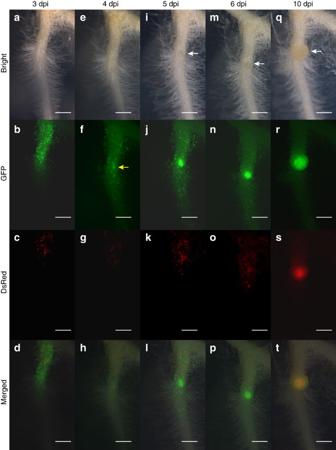Figure 4: Temporal and spatial expression ofpEpr3:tYFP-NLSactivity in Gifu. Time series on the same root from 3 to 10 dpi withM. lotiMAFF303099 DsRed.a–dare 3 dpi, (e–h) 4 dpi, (i–l) 5 dpi, (m–p) 6 dpi and (q–t) 10 dpi. (a,e,i,m,q) Bright-field images, (b,f,j,n,r) GFP filter images and (c,g,k,o,s) DsRed filter images. (d,h,l,p,t) Merged bright, GFP and DsRed images. White arrows indicate nodule development and yellow arrow indicate strongpEpr3:tYFP-NLSexpression in the epidermal cell in response toM. loti. Scale bars, 0.5 mm. Figure 4: Temporal and spatial expression of pEpr3:tYFP-NLS activity in Gifu. Time series on the same root from 3 to 10 dpi with M. loti MAFF303099 DsRed. a – d are 3 dpi, ( e – h ) 4 dpi, ( i – l ) 5 dpi, ( m – p ) 6 dpi and ( q – t ) 10 dpi. ( a , e , i , m , q ) Bright-field images, ( b , f , j , n , r ) GFP filter images and ( c , g , k , o , s ) DsRed filter images. ( d , h , l , p , t ) Merged bright, GFP and DsRed images. White arrows indicate nodule development and yellow arrow indicate strong pEpr3:tYFP-NLS expression in the epidermal cell in response to M. loti . Scale bars, 0.5 mm. 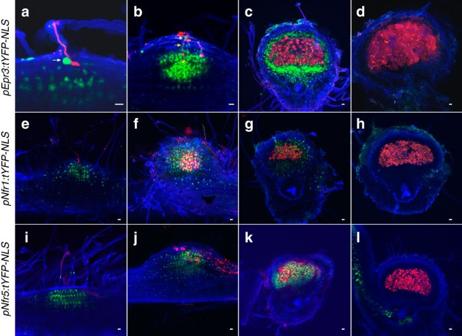Figure 5: Temporal and spatial expression ofEpr3andNfrpromoter reporter constructs. Images of the infection process from the root hair infection stage (a,e,i) to nodule maturity (d,h,l) were collected from sections/whole mounts of transgenic roots inoculated withM. lotiMAFF303099 DsRed. (a–d)pEpr3:tYFP-NLS, (e–h)pNfr1:tYFP-NLSand (i–l)pNfr5:tYFP-NLS. White and yellow arrows show specificEpr3expression in epidermal and outer cortical cells adjacent to infection threads. Scale bars, 20 μm. Full size image Figure 5: Temporal and spatial expression of Epr3 and Nfr promoter reporter constructs. Images of the infection process from the root hair infection stage ( a , e , i ) to nodule maturity ( d , h , l ) were collected from sections/whole mounts of transgenic roots inoculated with M. loti MAFF303099 DsRed. ( a – d ) pEpr3:tYFP-NLS , ( e – h ) pNfr1:tYFP-NLS and ( i – l ) pNfr5:tYFP-NLS . White and yellow arrows show specific Epr3 expression in epidermal and outer cortical cells adjacent to infection threads. Scale bars, 20 μm. Full size image Previous results showed that Epr3 expression was rapidly induced in the epidermal cells after Nod factor application or rhizobia inoculation [57] . Considering the developmental expression pattern of Epr3 described above, we asked whether Nfr1 , Nfr5 and Epr3 would be co-expressed and hence whether Nfr1 and Nfr5 could be involved in the cellular regulation in both root epidermis and cortex. First, pEpr3:GUS was transformed into nfr1 and nfr5 mutants to assay Epr3 promoter activation. The absence of reporter gene activity in these genotypes shows that Epr3 promoter activation is dependent on both Nfr1 and Nfr5 ( Fig. 6c ; Supplementary Table 1 ). Second, the expression of Nfr1 and Nfr5 was monitored using promoter GUS reporters. Both promoters were active in uninoculated root epidermal cells, as expected for Nod factor receptors ( Supplementary Fig. 2g,k ). Additional detailed studies using pNfr1:tYFP-NLS and pNfr5:tYFP-NLS constructs confirmed whole root expression in the uninoculated roots ( Supplementary Fig. 3 ). The Nfr1 promoter was generally found to have a lower level of activity compared to Nfr5 . In inoculated roots, the Nfr1 and Nfr5 promoters remained active within infected root hairs, but activity of the Nfr1 promoter was difficult to detect using the tYFP-NLS and GUS fusion constructs due to the low expression level ( Fig. 5e ; Supplementary Fig. 2h,l ). At later time points, this epidermal expression weakened and was followed by expression in the cortex as the development of nodule primordia progressed. No Epr3 , Nfr1 or Nfr5 promoter activity was observed in fully developed nodules ( Fig. 5d,h,l ; Supplementary Fig. 2e,j,m ). 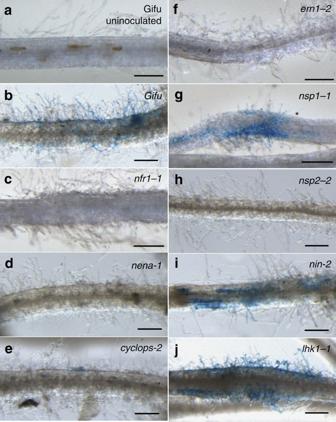Figure 6:Epr3promoter activation and transcript levels in symbiotic mutants. Images of transgenic roots stained forpEpr3:GUSactivation in Gifu and symbioticLotusmutants inoculated with R7A and assayed 3–10 dpi. (a) Uninoculated Gifu control (b), inoculated Gifu, (c)nfr1-1, (d)nena-1, (e)cyclops-2, (f)enr1-2, (g)nsp1-1, (h)nsp2-2(i)nin-2and (j)lhk1-1. Scale bars, 250 μm. SeeSupplementary Table 1for the complete data set and the number of plants analysed. Figure 6: Epr3 promoter activation and transcript levels in symbiotic mutants. Images of transgenic roots stained for pEpr3:GUS activation in Gifu and symbiotic Lotus mutants inoculated with R7A and assayed 3–10 dpi. ( a ) Uninoculated Gifu control ( b ), inoculated Gifu, ( c ) nfr1-1 , ( d ) nena-1 , ( e ) cyclops-2 , ( f ) enr1-2 , ( g ) nsp1-1 , ( h ) nsp2-2 ( i ) nin-2 and ( j ) lhk1-1 . Scale bars, 250 μm. See Supplementary Table 1 for the complete data set and the number of plants analysed. Full size image These results show that both Nfr1 and Nfr5 are expressed in the cells, where Epr3 is induced in the root cortex. This suggests that the two-step recognition signalling mediated by Nod factor and EPS perception by LysM receptor proteins at the epidermal root interface may also be operative in the cortical cell layers and in nodule primordia as the rhizobial infection progresses. Symbiotic transcription factors coordinate Epr3 expression Studies in Lotus and Medicago have contributed to the understanding of a symbiotic signal transduction pathway acting downstream of the Nod factor receptors [59] . Activation of this pathway is critical for initiating infection and/or organogenesis [7] . We took advantage of available loss-of-function mutants inactivating these pathways and the pEpr3:GUS reporter to examine whether Epr3 was independently regulated or integrated into these pathways ( Fig. 6 ). Initially, the role of genes primarily required for infection thread formation and/or progression was investigated in cerberus , nap1 and pir1 mutants transformed with pEpr3:GUS . Reporter gene activity was detected at levels and locations similar to Gifu, indicating that these genes were not essential for Epr3 expression ( Supplementary Table 1 ). However, reporter gene expression driven by the Epr3 promoter was absent in mutants acting upstream of Ca 2+ spiking ( nfr1 , nfr5 , symrk , nup133 , pollux and nena ) and in ccamk mutants impaired in their ability to interpret the calcium oscillations ( Fig. 6 ; Supplementary Table 1 ). Nod factor perception and the onset and interpretation of Ca 2+ spiking through the common symbiosis pathway were thus required for Epr3 activation. Similar analyses in mutants lacking symbiotic transcriptional activators revealed a differential genetic requirement for the epidermal and cortical onset of Epr3 transcription. We found no detectable epidermal expression in nsp2 and ern1 mutants, a very reduced expression in cyclops , while Nsp1 and Nin were dispensable for epidermal expression ( Fig. 6 ). Further evidence for differential regulation of Epr3 expression in the epidermal and cortical primordia was obtained from nena , cyclops , nsp1 and ern1 mutants, which eventually initiate the organogenesis program in the cortical layers leading to nodule primordia formation, and from the snf1 mutant (CCaMK gain of function; Supplementary Fig. 4 ; Supplementary Table 1 ). In these mutants, the Epr3 promoter was active in the emerging nodule primordia. We then investigated whether promoter sequences mediating epidermal and cortical Epr3 expression could be delimited in transgenic Gifu roots using a set of promoter deletions. In these Gifu roots, the 1,019 (ref. 57 ), 684, 329 and 280 bp promoters induced GUS expression in both the epidermis and nodule primordia. However, further deletion of promoter sequences to 257 bp eliminated epidermal expression while activation in nodule primordia was still observed ( Fig. 7a,c ). This analysis positions a regulatory promoter element sufficient for epidermal expression between 280 and 257 bp, and an element regulating primordial expression within the 257 bp promoter. Mutation of a sequence in the 280 bp promoter segment (mutation 1) corresponding to a previously characterized AP2 transcription factor binding site [60] eliminates epidermal Epr3 expression ( Fig. 7b,c ). In contrast, no detectable change in epidermal expression was observed after mutation of a sequence corresponding to a previously identified NIN-binding site [39] , [61] in the 280 promoter (mutation 2). However, mutation of this NIN1-binding site in the 257 bp promoter eliminates the cortical expression ( Fig. 7b,c ), suggesting that ERN1 can still activate the Epr3 280 promoter lacking the NIN1-binding site (mutation 2) in the cortex. The role of the predicted ERN1- and NIN1-binding sites of the 280 bp Epr3 promoter segment ( Fig. 7b ) was further investigated in an electrophoretic mobility shift assay (EMSA; Fig. 7f ). Full-length ERN1 and truncated NIN (residues 520–878) proteins were expressed in Escherichia coli and binding of DNA probes encompassing the corresponding binding sites was determined as mobility shifts ( Fig. 7b,f ; Supplementary Table 2 ). Mobility shifts were observed for both the ERN1 and NIN proteins, and binding of DNA fragments carrying mutations found to impair epidermal or cortical expression in pEpr3:GUS analyses was eliminated or reduced ( Fig. 7f ). 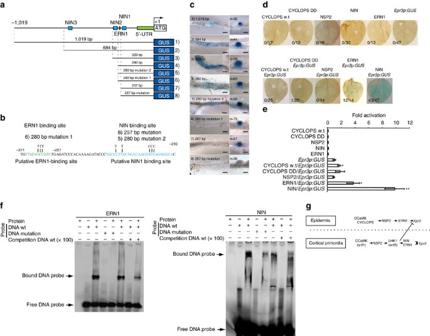Figure 7:Epr3promoter analysis in Gifu. (a) Overview of theEpr3promoter region and the analysed deletion series. Positions of three putative NIN-binding sites and one putative ERN1-binding site are indicated. (b) Nucleotide changes in the mutated putative binding sites for ERN1 and NIN. (c) Gifu plants transformed withpEpr3:GUSpromoter deletions were inoculated with R7A and assayed at 4–10 dpi. Panels showEpr3expression in epidermal and cortical cells. Scale bars, 0.5 mm. (d) ThepEpr3:GUS, and/or constructs for overexpression ofCyclops,Cyclops DD,Nsp2,Ern1andNinwere infiltrated intoN. benthamianaleaves. Upper row shows single infiltration, and bottom row is co-infiltration ofpEpr3:GUStogether with CYCLOPS, CYCLOPS DD, NSP2 or NIN. After 3 days incubation, these leaves were stained by X-gluc, and destained. Numbers indicate fraction of GUS-positive leaves. (e) Levels of GUS activity induced bypEpr3:GUSinN. benthamianaleaves after 3 days infiltration. Panel shows fold change compared topEpr3:GUSsingle infiltration. Error bars are s.e. * or ** (P<0.05 orP<0.01, Student’st-test,n=4–5) indicates significant difference compared topEpr3:GUSsingle infilutaration. (f) EMSAs were performed using His-tagged ERN1 and truncated NIN (residues 520–878) together with putative ERN1- and NIN-binding DNA sequences. Sequences of DNA wt and mutant versions of theEpr3promoter corresponds tob, and DNA probes were FAM-tagged. Competition DNA is 100 times concentration of wt DNA without FAM. (g) Model ofEpr3induction. In the epidermis, ERN1 is sufficient forEpr3expression downstream of CCaMK, CYCLOPS and NSP2. In the cortical primordia, both NIN and ERN1 induceEpr3expression directly downstream of CCaMK, NSP2 and the LHK1 cytokinin receptor. Cytokinin signaling through LHK1 has a negative effect on epidermalEpr3expression possibly involving the mechanism regulating infection thread formation43. Figure 7: Epr3 promoter analysis in Gifu. ( a ) Overview of the Epr3 promoter region and the analysed deletion series. Positions of three putative NIN-binding sites and one putative ERN1-binding site are indicated. ( b ) Nucleotide changes in the mutated putative binding sites for ERN1 and NIN. ( c ) Gifu plants transformed with pEpr3:GUS promoter deletions were inoculated with R7A and assayed at 4–10 dpi. Panels show Epr3 expression in epidermal and cortical cells. Scale bars, 0.5 mm. ( d ) The pEpr3:GUS , and/or constructs for overexpression of Cyclops , Cyclops DD , Nsp2 , Ern1 and Nin were infiltrated into N. benthamiana leaves. Upper row shows single infiltration, and bottom row is co-infiltration of pEpr3:GUS together with CYCLOPS, CYCLOPS DD, NSP2 or NIN. After 3 days incubation, these leaves were stained by X-gluc, and destained. Numbers indicate fraction of GUS-positive leaves. ( e ) Levels of GUS activity induced by pEpr3:GUS in N. benthamiana leaves after 3 days infiltration. Panel shows fold change compared to pEpr3:GUS single infiltration. Error bars are s.e. * or ** ( P <0.05 or P <0.01, Student’s t -test, n =4–5) indicates significant difference compared to pEpr3:GUS single infilutaration. ( f ) EMSAs were performed using His-tagged ERN1 and truncated NIN (residues 520–878) together with putative ERN1- and NIN-binding DNA sequences. Sequences of DNA wt and mutant versions of the Epr3 promoter corresponds to b , and DNA probes were FAM-tagged. Competition DNA is 100 times concentration of wt DNA without FAM. ( g ) Model of Epr3 induction. In the epidermis, ERN1 is sufficient for Epr3 expression downstream of CCaMK, CYCLOPS and NSP2. In the cortical primordia, both NIN and ERN1 induce Epr3 expression directly downstream of CCaMK, NSP2 and the LHK1 cytokinin receptor. Cytokinin signaling through LHK1 has a negative effect on epidermal Epr3 expression possibly involving the mechanism regulating infection thread formation [43] . Full size image Elevated cytokinin levels and signalling have been shown to regulate the number of infection threads progressing into the root cortex [43] , [62] . We asked whether Epr3 expression would be regulated by cytokinin signalling. Gifu roots were treated with 10 −8 M BAP and the Epr3 transcript was quantified after 3, 6 or 12 h. In contrast to Nod factor treatment, application of cytokinin did not induce detectable Epr3 expression in roots during this short-term treatment ( Supplementary Fig. 5a ), while Epr3 was expressed in spontaneous nodule primordia formed by snf2 ( Supplementary Fig. 4h,i ). Additional insight into the role of cytokinin signalling on Epr3 expression was obtained from the analysis in the loss-of-function cytokinin receptor lhk1-1 mutant. In the lhk1-1 genetic background, the Epr3 :GUS activity was abundant in the root hairs/epidermis compared to wild type, at the same time point after inoculation ( Fig. 6j ). Likewise, the overall Epr3 transcript level was higher in lhk1-1 mutant roots at 3 and 14 dpi compared to wild type ( Supplementary Fig. 5b,c ). This indicates that cytokinin signalling is, directly or indirectly, involved in repression of epidermal Epr3 expression and correlates the Epr3 expression level to the frequency of infection thread progression known to be increased in lhk1-1 mutants [43] . Our detailed analyses of the onset of Epr3 transcription in various symbiotic mutants revealed that the activation of the EPS recognition step has a differential genetic requirement in the epidermal cell layer, compared to the root cortex where nodule primordia emerge. The increased Epr3 expression in lhk1-1 mutants and induction of Epr3 in primordia of snf2 mutants suggests that cytokinin signalling has opposing effects on Epr3 expression in epidermal and cortical cells. Promoter elements mediate cell layer-specific expression Analysis of genetic requirements for Epr3 promoter activation during root nodule symbiosis revealed that CYCLOPS, NSP2 and ERN1 transcriptional regulators control Epr3 expression in epidermal root cells. To assess whether this control is exerted through Epr3 promoter elements, Epr3 promoter activation was investigated by transient co-expression in Nicotiana benthamiana leaves. Constructs expressing CYCLOPS or the autoactive DD version of CYCLOPS [31] previously shown to activate Nin expression were infiltrated into N. benthamiana leaves together with pEpr3:GUS . Epr3 promoter activation was monitored by staining leaves for GUS activity ( Fig. 7d,e ). GUS activity was comparable to that of pEpr3:GUS alone after co-infiltration of CYCLOPS or the autoactive DD version. Similarly, co-expression of an NSP2 construct and pEpr3:GUS did not result in detectable Epr3 promoter activation. In contrast, co-infiltration of ERN1 and pEpr3:GUS resulted in expression of the Epr3 promoter ( Fig. 7d,e ). A previous report indicated that Epr3 is downstream of Nin [39] , [63] while our promoter studies suggested this may only be the case for cortical Epr3 expression. However, lack of primordia in nin mutants prevented detection of pEpr3:GUS- based assessment of NIN involvement in cortical expression of Epr3 . A construct expressing NIN was therefore infiltrated into N. benthamiana leaves together with pEpr3:GUS and was able to activate the Epr3 promoter ( Fig. 7d,e ). These results suggest that ERN1 is essential for Epr3 expression in both epidermal and cortical cells and delimits an ERN1-binding site mediating epidermal expression of Epr3 in the epidermis. NIN is essential for induction of Epr3 expression in cortical cells ( Fig. 7g ) and a NIN1-binding site sufficient for cortical cell expression was delimited in the Epr3 promoter. The deletion study did not reveal a major contribution from the putative NIN2- and NIN3-binding sites in the Epr3 promoter ( Fig. 7a ). Taken together, our results suggest that ERN1 is sufficient for epidermal Epr3 expression while NIN appears to be dependent on ERN1 for any epidermal regulation of Epr3 that may not have been uncovered by our promoter analysis. EPS perception leads to efficient symbiotic nodule formation The experiments monitoring the capacity of R7A to infect nodules of epr3 mutants revealed significant qualitative differences to wild-type Gifu. This prompted us to ask whether there were associated quantitative changes in nodulation efficiency. Nodule formation kinetics in Gifu and two allelic epr3 mutants, epr3-9 and epr3-11 , were determined after inoculation with R7A under standard conditions at 21 °C and the infection efficiency estimated from the number/ratio of pink versus white nodules ( Supplementary Fig. 6a ). A significant delay in infection efficiency resulting in mature nodules was detected in epr3-9 and epr3-11 compared to Gifu ( Supplementary Fig. 6a ). At 10 and 14 dpi, a significant reduction in infected pink nodules was observed on epr3-9 and epr3-11 plants compared with Gifu plants, while at 28 dpi, the number of pink nodules on epr3-9, epr3-11 and Gifu was comparable. To test whether this phenotypic change in infection efficiency was robust, the same experiment was performed at 28 °C. Nodulation of Gifu inoculated with R7A at 28 °C was reduced and delayed compared to 21 °C. However, the development of pink nodules on epr3-9 and epr3-11 was further delayed and reduced ( Supplementary Fig. 6a ). Similar results were obtained with MAFF303099, a highly infective M. loti strain ( Supplementary Fig. 6b ). Previously, a delay in the nodulation of Gifu at 21 °C was observed with the R7AexoB mutant strain that is unable to synthesize EPS [57] , [58] and this delay is exacerbated at 28 °C ( Supplementary Fig. 6c ) [57] . In contrast to R7A-inoculated Gifu plants, no pink nodules had developed by 28 dpi on R7AexoB-inoculated Gifu plants. Furthermore, R7AexoB-inoculated Gifu plants carried significantly fewer pink nodules and more white nodules than R7A-inoculated plants at 35 and 42 dpi. These results indicate that EPS and EPS perception by EPR3 are important for the timely progression of nodule infection and affect nodule development. We have shown that the EPR3 LysM receptor kinase perception of rhizobial EPS promotes proficient intracellular infection of root cortical cells and efficient symbiotic interaction between Lotus and M. loti . In contrast to the nfr1 and nfr5 Nod factor receptor mutants, which are strictly required for the initiation of nodulation [9] , [11] , [64] , epr3 mutants are nodulated and infected by M. loti , albeit with reduced efficiency and with a delay. The mutation of Epr3 or of EPS synthesis genes in the microbial partner reduces or eliminates nodule infection via infection threads and reduces the number of infected cells. Although a passive physicochemical contribution from EPS cannot be excluded, the phenotypic differences between epr3 mutants and wild-type plants inoculated with R7AexoB ( Supplementary Fig. 6 ) may suggest that EPR3 has a co-receptor that is partially functional in the absence of EPR3. Microscopy of root nodules shows that Epr3 is not only necessary for efficient intracellular infection across the epidermis but also in the root cortex and in nodule primordia. Inactivation of Epr3 results in a reduction of the normal intracellular infection thread mode and increased intercellular infection. Infection threads releasing bacteria between the primordial cells and crack entry both appear to contribute to the intercellular infection mode. One possibility is that in addition to promoting infection thread formation, EPR3 signalling plays a negative role in the control of crack entry and intercellular infection. In this scenario, a default intercellular infection pathway would take control when Epr3 is inactivated. Such a regulatory role is supported by the different phenotype of epr3 mutants compared to other infection thread mutants. In most of these developmental mutants, infection threads are arrested in the root hairs or misguided at the cortical boundary and little or no infection of primordia occurs [21] , [22] , [23] , [32] , [45] , [46] , [48] , [50] , [51] , [52] , [53] . The Nfr1 and Nfr5 Nod factor receptor genes are expressed in epidermal cells of uninoculated roots indicating the necessity for rapid and first-line perception of rhizobial signals by the legume root ( Supplementary Fig. 2g,k ; Supplementary Fig. 3 ) [11] . On the other hand, Epr3 expression is Nod factor-induced ( Supplementary Fig. 5a ) [57] , and Nfr1 - and Nfr5- dependent ( Fig. 6c ; Supplementary Table 1 ), positioning EPS-induced EPR3 signalling in a subsequent epidermal recognition step of a two-step surveillance mechanism. We show here that a spatially restricted increase in the expression of the Nod factor and EPS receptors occurs following the advancing symbiotic infection process. The Nfr1 , Nfr5 and Epr3 promoters are activated in root cortical zones where nodule primordia develop ( Fig. 5 ; Supplementary Fig. 2d,i,n ), a pattern also observed for SymRK and Lhk1 expression [42] , [65] , indicating receptor controlled signalling throughout rhizobia infection and primordia development. Taking into account that rhizobial nod genes are expressed in infection threads and that Nod factor synthesis is likely continuing during infection, this suggests that the two-step Nod factor and EPS recognition process assessing the compatibility of bacteria accompanies the progression of the infection thread from the epidermis into the cortical roots cells and nodule primordia. This interpretation is supported by the results obtained using a promoter with enriched epidermal activity to express Nfr1 in Lotus and Nfp (the Nfr5 homologue) in Medicago in their corresponding mutant backgrounds. In both experiments, cortical cell division was induced, but infection thread formation was restricted [8] , [66] . Furthermore, calcium spiking in the root cortex has been shown to follow the progressing infection thread [30] . Symbiotic mutant analyses in Lotus have allowed for the distinction of genes involved in the two pathways controlled by NFR1 and NFR5 following Nod factor perception, root hair infection and cortical organogenesis [7] . Our analysis reveals that Epr3 promoter activation takes place independently in both branches of the Nod factor signalling pathway and is dependent on genes acting before calcium spiking. Cyclops , Nsp2 and Ern1 , which control the root hair infection pathway [31] , [32] , [33] , [34] , [36] , [40] , [41] , [67] , also control early Epr3 activation ( Fig. 6 ), but not the later onset of transcription in cyclops and ern1 nodule primordia ( Supplementary Fig. 4 ). Epr3:GUS activation after co-expression in N. benthamiana and EMSAs suggest that ERN1 regulates Epr3 directly, while CYCLOPS and NSP2 act indirectly. The Epr3 promoter analyses suggest that Epr3 expression in the epidermis is regulated by ERN1. Furthermore, results from N. benthamiana leaves, using Epr3 short promoters and EMSA, indicate that both NIN and ERN1 control Epr3 in the cortex ( Fig. 7 ). Adding one more regulatory level, the fourfold increase in Epr3 transcript levels observed in the lhk1-1 mutant at 3 dpi and the increased epidermal expression of Epr3:GUS in lhk1-1 roots suggests that at early time points perception of cytokinin by LHK1 is important not only for controlling Nin levels [43] but also for the feedback regulation of Epr3 in the epidermal root hairs where infection threads are initiated ( Fig. 7g ). This feedback loop may involve ethylene as proposed for cytokinin regulation of infection thread formation [56] . Taken together, our results from the Epr3 transcriptional activation in both symbiotic pathways initiated downstream of calcium spiking corroborate with the observed effects of Epr3 mutations on infection. Thus, the results provide evidence for the role of this third LysM receptor during bacterial passage through the epidermis and subsequently during infection thread progression into the underlying cortical root tissues and nodule primordia. Plant material and growth conditions Lotus ecotype Gifu [68] was used as the wild-type plant. The epr3-9 and epr3-10 allels are single-nucleotide mutations, epr3-11 is a LORE 1 retrotransposon insertion [57] , [69] . For nodulations assays at 21 and 28 °C plants were grown in growth chambers (Sanyo MLR-351) with day/night cycles of 16/8 h. Plants were inoculated with OD 600 =0.02 bacterial suspensions. Bacterial strains and growth conditions Wild-type Mesorhizobium loti strains R7A (refs 70 , 71 ) and MAFF303099 (ref. 72 ) along with the EPS mutant R7AexoB [57] , [58] were grown in TY/YMB medium at 28 °C. DsRed-tagged strains were used in microscopy experiments [57] , [58] , [73] . Agrobacterium rhizogenes strains AR12 or AR1193 (refs 74 , 75 ) were used for all hairy root transformation experiments [76] . Agrobacterium tumefaciens strain AGL1 was used in N. benthamiana infiltration experiments. The following concentrations of antibiotics were used for M. loti and Agrobacterium strains: ampicillin, 100 μg ml −1 ; tetracycline, 2–10 μg ml −1 ; gentamicin, 50 μg ml −1 ; rifampicin, 100 μg ml −1 ; spectinomycin, 100 μg ml −1 ; and neomycin, 100 μg ml −1 and carb, 100 μg ml −1 for A. tumefaciens AGL1. Microscopy Nodules for light and TEM were embedded and sectioned [7] . Semi-thin nodule sections (5 μm) for light microscopy and ultra-thin (70 nm) sections for TEM were sliced using a Leica UCT ultramicrotome. Confocal microscopy of cortical infection threads was performed by hand-slicing 2-week-old nodules that were then stained with 0.04% Calcofluor White M2R (Fluorescent Brightener 28; Sigma). The cell wall and cortical infection threads were detected using a 410–490 nm filter, and M. loti DsRed were detected using a 587–665 nm filter on a Zeiss LSM 710 confocal microscope. For pEpr3:tYFP-NLS, pNfr1:tYFP-NLS and pNfr5:tYFP-NLS analysis, roots and nodule sections were prepared by hand-sectioning and nuclear fluorescence was observed using a 491–535 nm filter on a Zeiss LSM 710 confocal microscope. GUS staining Lotus roots were stained with 0.5 mg ml −1 5-bromo-4-chloro-3-indolyl-β- D -glucuronic acid, 100 mM potassium phosphate buffer (pH7.0), 1 mM potassium ferricyanide, 1 mM potassium ferrocyanide and 0.1% Triton X-100. Lotus roots were incubated at 21 °C overnight. Promoter and expression constructs pEpr3:tYFP-NLS and pEpr3:GUS full-length promoters [57] were used. Shortened Epr3 promoter regions (684 bp, 329 bp, 280 bp, 280 bp a mutated in ERN1-binding site, 280 bp a mutated in NIN1-binding site, 257 bp and 257 bp a mutated in NIN1-binding site) and the full-length Nsp2 gene were amplified by PCR and recombined into pDONR207 (Invitrogen) using the Gateway BP reaction (Invitrogen). These entry vectors were recombined into pIV10:GW:GUS and pCAMBIA1300:Ljubiquitin promoter:GW [77] destination vectors using Gateway LR reactions (Invitrogen). The Nfr1 promoter (4,171 bp) and terminator (394 bp) regions, and for Nfr5 , promoter (1,327 bp) and terminator (444 bp) have been used for building the pNfr1:GUS, pNfr1:tYFP-NLS , pNfr5:GUS, pNfr5:tYFP-NLS transcriptional reporter constructs. The resultant constructs were transformed into A. rhizogenes strain AR1193 and A. tumefaciens strain AGL1. See Supplementary Table 2 for primer sets. Epr3 induction analysis using N. benthamiana A. tumefaciens strain AGL1 transformed with appropriate vectors was grown in LB medium overnight. Cell pellets were collected by centrifugation and resuspended in 10 mM MgCl 2 , 10 mM MES (pH 6.5) and 0.15 mM acetosyringone. Suspensions were diluted to: OD 600 =0.1 for pEpr3:GUS , OD 600 =0.4 for pUbi:Nin , pUbi:Nsp2 , p35S:Cyclops , p35S:Cyclops DD and mixed with OD 600 =0.05 A. tumefaciens expressing the silencing suppressor p19. The mixed cultures were infiltrated into 4-week-old N. benthamiana leaves and 3 days later, leaves were collected and stained as described in the GUS-staining section at 37 °C overnight. After staining, leaves were decolorized using a 1:1:3 acetic acid:glycerol:ethanol solution at 65 °C twice for 1 h. GUS activity was quantified using 4-MUG [78] and fluorescence at 365 nm was measured on a Varian Cary Eclipse Fluorescence Spectrophotometer (Agilent). Quantitative PCR with reverse transcription gene expression analysis Nod factor and BAP were applied to roots and gene expression analysed [79] . For gene expression analysis in nin-2 and lhk1-1 mutants 10 plants were grown on ¼ B&D plates and inoculated with M. loti MAFF303099 or water (mock) at 14 or 3 days before collecting of roots. Three biological replicates were performed for each combination of mutant and time point. mRNA extraction, quality control checks and gene expression analysis using a Lightcycler480 instrument (Roche) [57] . Protein expression and purification The open reading frame corresponding to full-length ERN1 and NIN (residues 520–878) were cloned into the pET30 vector and proteins were expressed in E. coli LOBSTR cells [80] (Kerafast, Boston, USA). Bacterial cultures were grown at 37 °C to an optical density (OD600) of ∼ 0.6 and induced overnight with 0.2 mM isopropyl-β- D -thiogalactoside at 18 °C. Cells were opened by sonication in lysis buffer 1 for ERN1 (8 M urea, 25 mM Tris pH 7.8, 500 mM NaCl, 50 mM MgCl 2 , 10% glycerol and 30 mM imidazole) and in lysis buffer 2 for NIN (500 mM NaCl, 25 mM Tris pH 7.8 and 30 mM imidazole), supernatants were cleared by centrifugation, loaded onto Ni-sepharose 6 FF affinity resins (GE Healthcare) and extensively washed in their respective lysis buffers. ERN1 was refolded on the Ni-resin by adding native buffer (25 mM Tris pH 7.8, 500 mM NaCl, 50 mM MgCl 2 , 10% glycerol and 30 mM imidazole) following elution in the same buffer supplemented with 400 mM imidazole and NIN was eluted with lysis buffer 2 containing 400 mM imidazole. Electrophoretic mobility shift assay ERN1 and NIN were concentrated to 0.75 and 1.0 mg ml −1 , respectively, and mixed with (5(6)-Carboxyfluorescein) (FAM)-labelled promoter DNA segments ( Supplementary Table 2 ). DNA probes (final volum 25 nM) and 2 μl protein were incubated in binding buffer (25 mM Tris-HCl pH8.0, 80 mM NaCl, 35 mM KCl, 5 mM MgCl 2 , 10% (v/v) glycerol, 1 mM dithiothreitol and 0.1% (v/v) Triton100) for 30 min at 30 °C for ERN1 and 37 °C for NIN. These samples were subsequently separated in polyacrylamide gels (Criterion TGX Precast Gels; Bio-Rad) with 0.5 × TBE buffer at 80 V for 120 min. FAM fluorescence was detected using a Typhoon Trio (Amersham) Data availability The EPR3 sequence is available in Genebank, accession no. BAI79284.1. Other informational data are available within the manuscript file and its Supplementary Files or are available from the corresponding author upon request. How to cite this article: Kawaharada, Y. et al . Differential regulation of the Epr3 receptor coordinates membrane-restricted rhizobial colonization of root nodule primordia. Nat. Commun. 8, 14534 doi: 10.1038/ncomms14534 (2017). Publisher’s note: Springer Nature remains neutral with regard to jurisdictional claims in published maps and institutional affiliations.